A mechanical-force-driven physical vapour deposition approach to fabricating complex hydride nanostructures Nanoscale hydrides desorb and absorb hydrogen at faster rates and lower temperatures than bulk hydrides because of their high surface areas, abundant grain boundaries and short diffusion distances. No current methods exist for the direct fabrication of nanoscale complex hydrides (for example, alanates, borohydrides) with unique morphologies because of their extremely high reducibility, relatively low thermodynamic stability and complicated elemental composition. Here, we demonstrate a mechanical-force-driven physical vapour deposition procedure for preparing nanoscale complex hydrides without scaffolds or supports. Magnesium alanate nanorods measuring 20–40 nm in diameter and lithium borohydride nanobelts measuring 10–40 nm in width are successfully synthesised on the basis of the one-dimensional structure of the corresponding organic coordination polymers. The dehydrogenation kinetics of the magnesium alanate nanorods are improved, and the nanorod morphology persists through the dehydrogenation–hydrogenation process. Our findings may facilitate the fabrication of such hydrides with improved hydrogen storage properties for practical applications. Hydrogen-based energy is a promising means for solving the problems caused by the emission of greenhouse gases and depletion of fossil fuels [1] , [2] . However, the difficulties involved in ensuring safe, efficient and economical storage of hydrogen currently prevent hydrogen-based energy from being used practically. Hydrides can store hydrogen through solid-state chemical absorption and remain one of the most attractive groups for hydrogen storage because they deliver high gravimetric and volumetric densities [3] . Numerous efforts have been devoted to the exploration of hydride-based composites and high-performance catalysts towards the control of hydride thermodynamics, improvements in kinetics, and enhancements in recyclability [4] , [5] , [6] . Unfortunately, the technical requirements established for practical hydride applications have not yet been met. Complex hydrides, such as alanates and borohydrides, have recently attracted considerable interest as potential hydrogen storage materials [7] , [8] . However, their thermodynamics and kinetics are not appropriate for cycling under moderate pressure or temperature conditions. Nanoscale hydrides, with their high surface areas, abundant grain boundaries and short diffusion distances, have been shown to desorb and absorb hydrogen at faster rates and lower temperatures than bulk hydrides [9] , [10] . The conventional technique for preparing nanoscale hydrides is high-energy ball milling, which mechanically decreases the particle size. However, this top-down method generates a broad particle size distribution, where the smallest attainable particle size is approximately 100 nm although the crystallite size can typically be decreased to a few nanometres [11] , [12] , [13] , [14] . Such particles are usually inadequate to produce a significant size effect [15] . Nanoconfinement is a more recently developed strategy that creates smaller, more uniform nanoscale hydrides, typically through the infiltration of scaffolds with hydrides. This bottom-up approach has been successfully utilised to generate nanoconfined ammonia borane, alanates, borohydrides and magnesium hydrides within mesoporous silicas, nanostructured carbons and metal–organic frameworks [16] , [17] , [18] , [19] , [20] , [21] , [22] , [23] , [24] . Magnesium nanocrystals incorporated into a polymer (poly(methyl methacrylate)) display high hydrogen density (up to 6 wt% of Mg) and rapid kinetics (loading times <30 min at 200 °C) [18] . The temperature at the maximum desorption rate of 2–10 nm NaAlH 4 supported on carbon nanofibres is decreased to 70 °C [20] . Moreover, the desorption of hydrogen from nano-NaAlH 4 confined within the metal–organic framework material MOF-74(Mg) begins at 50 °C, nearly 100 °C lower than the temperature for bulk NaAlH 4 (ref. 22 ). Nano-LiBH 4 embedded in Ni-doped porous carbon absorbs approximately 10 wt% H 2 (versus LiBH 4 ) at 320 °C under 40 bar of H 2 , exhibiting a significantly improved hydrogen storage reversibility [23] . However, the dead weight contributed by the scaffold reduces the practical hydrogen storage capacity of the material to an unacceptable value. Moreover, in some respects, the confinement in the scaffolding environment makes it more difficult to understand and characterise the fundamental properties of the nanoscale hydrides. Several alternative bottom-up methods have also been proposed to prepare nanoscale hydrides without scaffolds or supports, including solution-based synthesis and thermal vapour deposition [25] , [26] , [27] , [28] , [29] . To the best of our knowledge, these methods are only available for MgH 2 , however, and are unfit for preparing nanoscale complex hydrides because of their extremely high reducibility, relatively low thermodynamic stability and complicated elemental composition. Therefore, exploring and developing novel synthesis methods for the preparation and stabilisation of nanoscale complex hydrides with unique morphologies and without the use of a scaffold are major challenges to the success of ‘nano-tuning’ strategies. In particular, this technique may also provide new opportunities for achieving improved hydrogen storage properties for practical applications. In this work, we present a novel, facile method called mechanical-force-driven physical vapour deposition (MFPVD), which can be followed with a low-temperature heat treatment, for the preparation of nanoscale complex hydrides. This technique was discovered serendipitously while investigating the effects of ball milling [Mg(AlH 4 ) 2 (Et 2 O)] n (Et 2 O: diethyl ether) on the hydrogen storage properties of Mg(AlH 4 ) 2 . It capitalises on the one-dimensional structure of the organic coordination polymer of complex hydrides. As a proof of principle, Mg(AlH 4 ) 2 nanorods measuring 20–40 nm in diameter and LiBH 4 nanobelts measuring 10–40 nm in width were successfully prepared for the first time. The dehydrogenation kinetics of the Mg(AlH 4 ) 2 nanorods were improved, and the nanorod morphology persisted throughout the dehydrogenation and hydrogenation processes. Such a technique is general enough to prepare nanostructures of other complex hydrides with one-dimensional organic coordination polymers containing removable ligands. 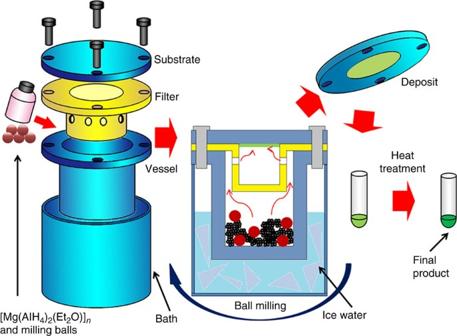Figure 1: A schematic diagram of the Mg(AlH4)2nanorod preparation process. First, raw [Mg(AlH4)2(Et2O)]nwas high-energy ball milled in a specially designed jar equipped with a filter, substrate and ice-water bath; this step led to the formation of a deposit on the substrate. The final product was obtained by heat-treating this deposit under vacuum at 90 °C. Synthesis and characterisation of nano-Mg(AlH 4 ) 2 and -LiBH 4 Figure 1 presents a schematic diagram of Mg(AlH 4 ) 2 nanorod preparation. Raw [Mg(AlH 4 ) 2 (Et 2 O)] n was ball milled at high energy in a specially designed jar, using a filter, substrate and ice-water bath to bring about deposit formation on the substrate. Subsequently, the final product was obtained by heat-treating the deposited material under vacuum at 90 °C. The sample phases were identified at different stages during preparation using X-ray diffraction (XRD) ( Fig. 2a ) and Fourier-transform infrared spectroscopy (FTIR) ( Fig. 2b ). The raw [Mg(AlH 4 ) 2 (Et 2 O)] n exhibited the same XRD pattern and FTIR spectrum as previously reported [30] . No diffraction peaks were visible in the XRD profile of the deposit, although the FTIR spectrum was nearly identical to that of the precursor, suggesting that the resulting deposit is amorphous [Mg(AlH 4 ) 2 (Et 2 O)] n . After performing the low-temperature heat treatment, only Mg(AlH 4 ) 2 diffraction peaks were visible in the XRD profile, and the C–H and C–O–C bands in the FTIR spectrum disappeared, while the Al–H band underwent a blue shift. In combination, these observations indicate the removal of Et 2 O from the system and the formation of Mg(AlH 4 ) 2 . The Rietveld fits to the diffraction patterns further supported this interpretation ( Supplementary Fig. 1 ). Scanning electron microscope imaging revealed that all the three samples had rod-like morphologies ( Fig. 2c–e ). Microrods measuring approximately 1 μm in diameter were observed for the raw [Mg(AlH 4 ) 2 (Et 2 O)] n ( Fig. 2c ), and encouragingly, uniform nanorods with diameters ranging from 20 to 40 nm were formed for both the deposit and final product ( Fig. 2d,e ). However, a small quantity of undesirable particles was also visible in these materials ( Supplementary Fig. 2 ), the reason for which is discussed later. On the basis of these results, we conclude that the high-energy ball milling of raw [Mg(AlH 4 ) 2 (Et 2 O)] n microrods deposited [Mg(AlH 4 ) 2 (Et 2 O)] n nanorods onto the substrate and that the Et 2 O molecules were liberated from the [Mg(AlH 4 ) 2 (Et 2 O)] n nanorods during subsequent heat treatments, forming the resulting Mg(AlH 4 ) 2 nanorods. The yield of Mg(AlH 4 ) 2 nanorods was determined to be approximately 40% in the present study. Figure 1: A schematic diagram of the Mg(AlH 4 ) 2 nanorod preparation process. First, raw [Mg(AlH 4 ) 2 (Et 2 O)] n was high-energy ball milled in a specially designed jar equipped with a filter, substrate and ice-water bath; this step led to the formation of a deposit on the substrate. The final product was obtained by heat-treating this deposit under vacuum at 90 °C. 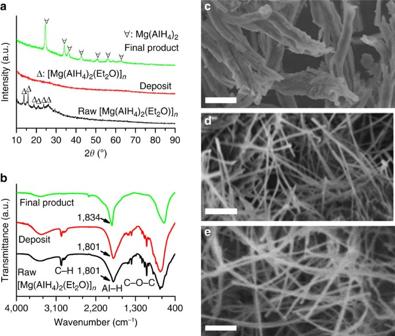Figure 2: Characterisations of the Mg(AlH4)2samples at different stages. (a) XRD patterns. A pure Mg(AlH4)2sample was obtained after MFPVD followed by low-temperature heat treatment. (b) FTIR spectra. After carrying out the heat treatment at 90 °C, the Al–H vibration characteristic to Mg(AlH4)2appeared at 1,834 cm−1, while the C–H and C–O–C bands were absent. s.e.m. images of (c) the raw [Mg(AlH4)2(Et2O)]n; (d) the deposit; (e) the resultant product. Scale bar in (c), 2 μm; scale bar in (d,e), 200 nm. Mg(AlH4)2nanorods ranging from 20 to 40 nm in diameter were obtained as the resulting product. a.u., arbitrary unit. Full size image Figure 2: Characterisations of the Mg(AlH 4 ) 2 samples at different stages. ( a ) XRD patterns. A pure Mg(AlH 4 ) 2 sample was obtained after MFPVD followed by low-temperature heat treatment. ( b ) FTIR spectra. After carrying out the heat treatment at 90 °C, the Al–H vibration characteristic to Mg(AlH 4 ) 2 appeared at 1,834 cm −1 , while the C–H and C–O–C bands were absent. s.e.m. images of ( c ) the raw [Mg(AlH 4 ) 2 (Et 2 O)] n ; ( d ) the deposit; ( e ) the resultant product. Scale bar in ( c ), 2 μm; scale bar in ( d , e ), 200 nm. Mg(AlH 4 ) 2 nanorods ranging from 20 to 40 nm in diameter were obtained as the resulting product. a.u., arbitrary unit. Full size image To demonstrate the general applicability of this method, a second experiment was performed using [LiBH 4 (MTBE)] n (MTBE: methyl tert -butyl ether) as the starting material for the preparation of LiBH 4 nanostructures. Ball milling was conducted on a planetary ball mill with a dry-ice bath. The deposit was evacuated at room temperature to remove the MTBE molecules. The morphology of the resulting product was observed using a JEM-2100 transmission electron microscope (TEM) equipped with a vacuum-transfer holder because nanoscale LiBH 4 is highly moisture sensitive. As shown in Fig. 3a , LiBH 4 nanobelts with widths of 10–40 nm were successfully obtained. The high-resolution (HR) image in Fig. 3b displays fringes with interplanar spacings of 0.37 nm, which corresponds to the separations between the (0 1 1) planes of LiBH 4 . No specific signals were detected in the spectrum obtained with energy-dispersive X-ray spectroscopy (EDS) ( Fig. 3c ), indicating that the resulting nanobelts were composed of light elements (Z ⩽ 5), viz., LiBH 4 , which is sensible because [LiBH 4 (MTBE)] n was used as the raw material. In addition, a series of linear diffraction spots was observed in the selected-area electron diffraction (SAED) pattern; the corresponding interplanar spacing was calculated to be 0.37 nm ( Fig. 3d ), which agrees well with the HR image. These results demonstrate that LiBH 4 nanobelts measuring 10–40 nm in width were also successfully synthesised via the MFPVD method. 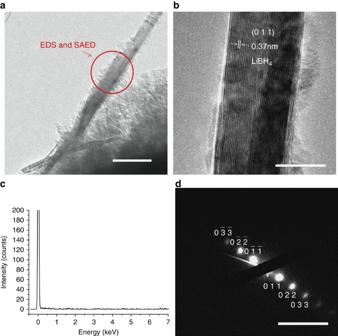Figure 3: Characterisations of LiBH4nanobelts. (a) TEM image of the LiBH4nanobelts. Scale bar, 50 nm. The red circle indicates the region examined by EDS and SAED. (b) HR image of the LiBH4nanobelts. Scale bar, 10 nm. (c) EDS spectrum of the marked region. (d) SAED pattern of the marked region. Scale bar, 10 nm−1. These results confirm the successful preparation of LiBH4nanobelts measuring 10–40 nm in width. Figure 3: Characterisations of LiBH 4 nanobelts. ( a ) TEM image of the LiBH 4 nanobelts. Scale bar, 50 nm. The red circle indicates the region examined by EDS and SAED. ( b ) HR image of the LiBH 4 nanobelts. Scale bar, 10 nm. ( c ) EDS spectrum of the marked region. ( d ) SAED pattern of the marked region. Scale bar, 10 nm −1 . These results confirm the successful preparation of LiBH 4 nanobelts measuring 10–40 nm in width. Full size image Hydrogen storage properties of nano-Mg(AlH 4 ) 2 and -LiBH 4 The hydrogen desorption behaviour of the Mg(AlH 4 ) 2 nanorods differed significantly from that of the bulk Mg(AlH 4 ) 2 (microrods of Mg(AlH 4 ) 2 (ref. 31 ), as shown in Fig. 4a . The thermal decomposition of the Mg(AlH 4 ) 2 microrods was carried out by a three-step reaction, and 6.7, 0.6 and 1.7 wt% of hydrogen were released during the progression of these three steps. In contrast, only two dehydrogenation steps were observed for the Mg(AlH 4 ) 2 nanorods in the temperature range tested. The hydrogen capacities of the first and second steps were 6.7 wt% and 2.3 wt%, respectively, while the total capacity remained 9.0 wt%. Evidently, after the particles reached nanoscale dimensions, the second and third Mg(AlH 4 ) 2 dehydrogenation steps merged. Notably, the dehydrogenation operating temperatures were decreased distinctly with the lowering of the onset and end temperatures by 30 °C and 80 °C, respectively. Moreover, the dehydrogenation rate of the Mg(AlH 4 ) 2 nanorods was significantly accelerated, as indicated in the isothermal dehydrogenation curves obtained at 120 °C ( Fig. 4b ). Approximately 4.7 wt% of hydrogen was released from the Mg(AlH 4 ) 2 nanorods within 30 min at 120 °C, while only 0.7 wt% of hydrogen was discharged from the microrods under the same conditions. The reaction kinetics observed during the second dehydrogenation stage of the Mg(AlH 4 ) 2 microrods and nanorods was compared further by first dehydrogenating the rods at 150 °C for 30 min and then rapidly heating them to 300 °C, followed by an isothermal hold for 1,500 s ( Supplementary Fig. 3 ). The Mg(AlH 4 ) 2 nanorods released approximately 78% of their hydrogen capacity within 500 s during the second dehydrogenation event. However, less than 10% of the available hydrogen was released from the Mg(AlH 4 ) 2 microrods under the same conditions. The apparent activation energy ( E a ) of the first dehydrogenation step was calculated via a Kissinger analysis [32] on the basis of the shifts in the maximum desorption rate ( T m ) with different heating rates ( β ). 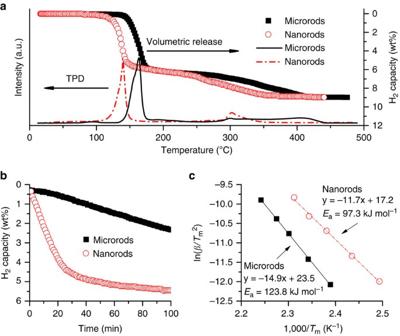Figure 4: Hydrogen desorption performance of Mg(AlH4)2microrods and nanorods. (a) TPD and volumetric release curves measured at 2 °C min−1. The Mg(AlH4)2nanorods exhibited a two-step dehydrogenation process with decreased operating temperatures. (b) Isothermal hydrogen desorption curves measured at 120 °C. Approximately 4.7 wt% of hydrogen was released from the Mg(AlH4)2nanorods within 30 min, while only 0.7 wt% was released for the microrods under the same conditions. (c) Kissinger plots. The apparent activation energy of the dehydrogenation decreased distinctly after the particles reached nanoscale dimensions. a.u., arbitrary unit. Figure 4: Hydrogen desorption performance of Mg(AlH 4 ) 2 microrods and nanorods. ( a ) TPD and volumetric release curves measured at 2 °C min −1 . The Mg(AlH 4 ) 2 nanorods exhibited a two-step dehydrogenation process with decreased operating temperatures. ( b ) Isothermal hydrogen desorption curves measured at 120 °C. Approximately 4.7 wt% of hydrogen was released from the Mg(AlH 4 ) 2 nanorods within 30 min, while only 0.7 wt% was released for the microrods under the same conditions. ( c ) Kissinger plots. The apparent activation energy of the dehydrogenation decreased distinctly after the particles reached nanoscale dimensions. a.u., arbitrary unit. Full size image In this study, the T m values were extracted from the non-isothermal volumetric release curves at β =1−10 °C min −1 ( Supplementary Fig. 4 ). By differentiating these curves, we obtained T m values of 127.9, 137.5, 146.8, 153.4 and 159.3 °C for heating rates of 1, 2, 4, 6, 10 °C min −1 , respectively. The values of E a was then determined from the slope of the ln( β / T m 2 ) versus 1/ T m . The resulting Kissinger plots ( Fig. 4c ) indicate that the E a values for the Mg(AlH 4 ) 2 microrods and nanorods were approximately 123.8 kJ mol −1 and 97.3 kJ mol −1 , respectively, revealing that the kinetic barrier for releasing hydrogen from the Mg(AlH 4 ) 2 nanorods was lower. The fully dehydrogenated samples were hydrogenated at elevated temperatures using an initial hydrogen pressure of 100 bar. The samples were gradually heated at 1 °C min −1 to a preset temperature and were subsequently held for 24 h. The hydrogenation curves of the fully dehydrogenated samples ( Fig. 5a ) reveal that the dehydrogenated Mg(AlH 4 ) 2 nanorods began absorbing hydrogen at 120 °C, which is 30 °C lower than the onset temperature of the microrods. However, only 2.3 wt% of hydrogen was absorbed by either sample, indicating improved but still partial hydrogenation of the nanorods. For the Mg(AlH 4 ) 2 nanorods, hydrogen uptake was completed within 150 s at 200 °C ( Fig. 5b ). The hydrogenation kinetics of the dehydrogenated Mg(AlH 4 ) 2 nanorods were superior to those of Mg nanowires with similar particle sizes [25] , [26] , [27] . Magnesium nanowires with diameters of 30–50 nm reportedly reached only 54% of their hydrogen-absorption capacity following 500 s of treatment at 200 °C [26] . Further cycling measurements identified good stability with 2.2 wt% reversible capacity of the dehydrogenated Mg(AlH 4 ) 2 nanorods over the first five cycles ( Fig. 5c ). Here, the slightly low hydrogen capacity was mainly attributed to the use of an insufficient holding time during the cycling measurements. 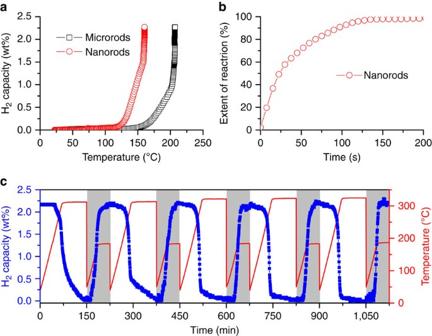Figure 5: Hydrogen-absorption and cycling performances of Mg(AlH4)2nanorods. (a) Hydrogenation curves of the fully dehydrogenated samples measured at 1 °C min−1. The dehydrogenated Mg(AlH4)2nanorods absorb approximately 2.3 wt% of hydrogen using a lower operating temperature than that required for the microrods. (b) Isothermal hydrogenation curve for the dehydrogenated nanorods measured at 200°C under 100 bar of hydrogen. The hydrogenation can be completed within 150 s. (c) Hydrogen desorption/absorption cycle curves. The grey regions denote 100 bar of hydrogen pressure, while the other regions denote vacuum. The Mg(AlH4)2nanorods exhibited good cycling stability with a 2.2 wt% reversible hydrogen capacity during the first five cycles. Figure 5: Hydrogen-absorption and cycling performances of Mg(AlH 4 ) 2 nanorods. ( a ) Hydrogenation curves of the fully dehydrogenated samples measured at 1 °C min −1 . The dehydrogenated Mg(AlH 4 ) 2 nanorods absorb approximately 2.3 wt% of hydrogen using a lower operating temperature than that required for the microrods. ( b ) Isothermal hydrogenation curve for the dehydrogenated nanorods measured at 200°C under 100 bar of hydrogen. The hydrogenation can be completed within 150 s. ( c ) Hydrogen desorption/absorption cycle curves. The grey regions denote 100 bar of hydrogen pressure, while the other regions denote vacuum. The Mg(AlH 4 ) 2 nanorods exhibited good cycling stability with a 2.2 wt% reversible hydrogen capacity during the first five cycles. Full size image In addition, a preliminary investigation of the dehydrogenation properties using temperature-programmed desorption (TPD) found apparent hydrogen release starting at around 60 °C for the as-prepared LiBH 4 nanobelts, however, no hydrogen release was detected for pristine LiBH 4 at such temperatures ( Supplementary Fig. 5 ). However, it was difficult to characterise accurately the hydrogen storage properties of the LiBH 4 nanobelts because of the relatively low yield obtained in this study. Further investigations on ways to increase the yield of LiBH 4 nanobelts are currently underway in our laboratory. Structural and morphological changes of nano-Mg(AlH 4 ) 2 The phase transformations and morphological changes that occurred during the Et 2 O removal and dehydrogenation processes were further investigated via in situ environmental TEM at elevated temperatures using an initial [Mg(AlH 4 ) 2 (Et 2 O)] n nanorod sample ( Supplementary Movie 1 ). 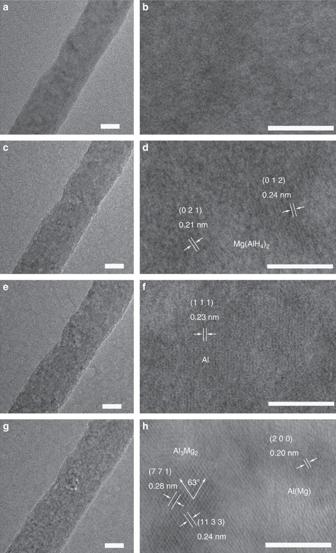Figure 6:In situTEM images of [Mg(AlH4)2(Et2O)]nnanorod at different stages. (a,b) Typical [Mg(AlH4)2(Et2O)]nnanorod at room temperature. (c,d) Nanorod after desorption at 100 °C; (e,f) desorption at 180 °C; (g,h) desorption at 400 °C. Scale bar in (a,c,e,g), 20 nm; scale bar in (b,d,f,h), 5 nm. The nanorod morphology persisted throughout the Et2O removal and dehydrogenation processes. Figure 6 displays the in situ environmental TEM images of [Mg(AlH 4 ) 2 (Et 2 O)] n nanorod samples, recorded at four different stages in the TPD curve ( Supplementary Fig. 6 ). We used an [Mg(AlH 4 ) 2 (Et 2 O)] n nanorod, with a diameter of 40 nm and a smooth surface at room temperature, as a representative specimen ( Fig. 6a ). The HR image revealed no observable lattice fringes, as shown in Fig. 6b , indicating that the nanorod was amorphous. The nanorod diameter remained constant following the removal of Et 2 O at 100 °C, while the nanorod surface became rough ( Fig. 6c ). Small Mg(AlH 4 ) 2 grains with interplanar spacings of either 0.21 or 0.24 nm, which correspond to the separations between the (0 2 1) and (0 1 2) planes, respectively, were identified from the fringes ( Fig. 6d ). Here, 100 °C was used as the Et 2 O-removal temperature instead of the value of 90 °C mentioned in the heat treatment described above because these in situ TEM measurements necessitate the use of higher heating rates and shorter holding times. After the first dehydrogenation event at 180 °C, the nanorod-like morphology persisted, and the surface roughness increased ( Fig. 6e ). Only Al grains, identified as the Al (1 1 1) planes, are visible in the HR image ( Fig. 6f ), while the XRD pattern ( Supplementary Fig. 7 ) reveals both Al and MgH 2 phases. A careful search in this region did not find the expected MgH 2 , possibly due to poor crystallinity. The specimen maintained its nanorod morphology when fully dehydrogenated at 400 °C ( Fig. 6g ). The HR image ( Fig. 6h ) identified the Al 3 Mg 2 (7 1 1) and (11 3 3) planes with a 63° angle and the Al(Mg) (2 0 0) planes. These observations were confirmed in the XRD pattern ( Supplementary Fig. 7 ). Therefore, the nanorod morphology was maintained throughout the two decomposition steps of Mg(AlH 4 ) 2 : Figure 6: In situ TEM images of [Mg(AlH 4 ) 2 (Et 2 O)] n nanorod at different stages. ( a , b ) Typical [Mg(AlH 4 ) 2 (Et 2 O)] n nanorod at room temperature. ( c , d ) Nanorod after desorption at 100 °C; ( e , f ) desorption at 180 °C; ( g , h ) desorption at 400 °C. Scale bar in ( a , c , e , g ), 20 nm; scale bar in ( b , d , f , h ), 5 nm. The nanorod morphology persisted throughout the Et 2 O removal and dehydrogenation processes. Full size image After hydrogenating the nanorods at 160 °C and a hydrogen pressure of 100 bar, the nanorods measuring 20–40 nm in diameter were also observed in scanning electron microscope and TEM images ( Supplementary Fig. 8 ). Moreover, the Al (2 0 0) and MgH 2 (1 0 1) planes were readily detectable in the HR image ( Supplementary Fig. 8c ), consistent with the XRD data ( Supplementary Fig. 9 ). These results indicate that the Mg(AlH 4 ) 2 nanorod morphology is also stable during hydrogenation, although only the second dehydrogenation step is reversible. Therefore, it is concluded that the nanorod-like morphology remained unchanged during the dehydrogenation and hydrogenation processes, despite involving complicated transformations with multiple phases. This finding demonstrates that nanoscale complex hydrides are durable during cycling even without nanoconfinement. As a result of this property, it can be said that nanoscale complex hydrides are superior to other well-known nanometre-sized particles, which tend to aggregate and form larger particles during thermal dehydrogenation and hydrogenation [11] , [14] . During the MFPVD process, the formation of the [Mg(AlH 4 ) 2 (Et 2 O)] n nanorods and [LiBH 4 (MTBE)] n nanobelts can be described as a vapour–solid growth mechanism. As previously reported [30] , [Mg(AlH 4 ) 2 (Et 2 O)] n is an organic coordination polymer that possesses a one-dimensional chain-like structure in which the [AlH 4 ] − tetrahedrons act as bridging units, with two rows of Et 2 O molecules shielding their edges. The [Mg(AlH 4 ) 2 (Et 2 O)] n chains in the lattice are separated by Et 2 O molecules and interact through weak van der Waals forces. During high-energy ball milling, the intense physical forces that are as high as several GPa at the collision points can easily destroy the van der Waals interactions, driving the raw [Mg(AlH 4 ) 2 (Et 2 O)] n into the vapour phase. The vaporised material eventually floats through the filter, deposits onto the substrate and self-assembles one-dimensionally according to its specific anisotropic molecular structure. This formation mechanism was confirmed by the failure encountered in the attempted preparation of Mg(AlH 4 ) 2 nanorods using both an Mg(AlH 4 ) 2 (THF) adduct and Mg(AlH 4 ) 2 as the starting materials, which lacked the one-dimensional molecular structure ( Supplementary Fig. 10 ). Low temperatures were maintained during the ball-milling procedure by using an ice-water bath to prevent the decomposition of [Mg(AlH 4 ) 2 (Et 2 O)] n . Occasionally, small particles may have passed through the filter and settled on the substrate, and formed the undesirable particles mentioned above. However, these contaminants could be avoided by future improvement to the filter. During successive low-temperature heat treatments, the Et 2 O molecules were removed without breaking the Al–H bonds, leading to the formation of Mg(AlH 4 ) 2 nanorods with an inherited one-dimensional morphology. This initial conjecture was supported by the successful preparation of LiBH 4 nanobelts with widths of 10–40 nm ( Fig. 3 ), via the MFPVD method using [LiBH 4 (MTBE)] n as the starting material, which also exhibits a one-dimensional chain-like structure [33] . It is therefore anticipated that this bottom-up approach can be extended to other complex hydrides with one-dimensional organic coordination polymers containing complex hydride groups and removable ligands [33] , [34] , [35] . In summary, we have developed a MFPVD procedure for the preparation of nanoscale complex hydrides without the use of a scaffold or support. As the prototypical complex hydrides, Mg(AlH 4 ) 2 nanorods with diameters of 20–40 nm and LiBH 4 nanobelts with widths of 10 nm–40 nm were successfully synthesised by the high-energy ball milling of [Mg(AlH 4 ) 2 (Et 2 O)] n and [LiBH 4 (MTBE)] n , respectively, followed by low-temperature heat treatment of the corresponding deposits. Our approach capitalises on the one-dimensional structure of the organic coordination polymers of complex hydrides. The hydrogen storage properties of the support-free Mg(AlH 4 ) 2 and LiBH 4 nanostructures obtained by this technique were superior to those of their bulk counterparts, and the Mg(AlH 4 ) 2 nanorod morphology persisted throughout the dehydrogenation and hydrogenation processes, suggesting good potential for reversible storage. The yield of these complex hydride nanostructures needs to be increased, however, before this technique can be used to obtain superior hydrogen storage properties for practical applications. Chemicals The [Mg(AlH 4 ) 2 (Et 2 O)] n and Mg(AlH 4 ) 2 microrods were prepared using the method described in our previous work [31] . LiBH 4 (95%, Sigma-Aldrich, USA) was used as received without further purification, and MTBE (AR-grade, Sinopharm, China) was distilled over sodium before use. All materials were handled and transferred either in a glove box (MBRAUN, Germany) filled with argon or under pure, flowing argon. High-energy ball milling A specially designed jar was used with the substrate, vessel and milling balls made of stainless steel, and with a filter made of nylon. For each experiment, 1 g of raw materials ([Mg(AlH 4 ) 2 (Et 2 O)] n or [LiBH 4 (MTBE)] n ) and 60 g of balls were loaded into the jar. High-energy ball milling was performed using a planetary ball mill (QM-3SP4, Nanjing, China) at 500 r.p.m. for 2 h. Ligand removal For the experiment involving [Mg(AlH 4 ) 2 (Et 2 O)] n , the temperature was raised to 90 °C at a heating rate of 2 °C min −1 , and then was held for 30 min under vacuum. For [LiBH 4 (MTBE)] n , the temperature was held at room temperature for 20 min under vacuum. Property evaluation TPD was performed using an online mass spectrometer (Hiden QIC-20, UK). Approximately 20 mg of each sample was loaded into a stainless-steel reactor and gradually heated from room temperature to 500 °C at a rate of 2 °C min −1 under continuously flowing pure Ar. The volumetric release and uptake results were assessed using a homemade Sieverts-type apparatus. The temperatures and pressures in the reactor and gas reservoir were monitored using thermoelectric couples and high-precision pressure transducers. The released hydrogen was quantified by calculating the pressure changes in the reactor using the equation of state. Structural characterisation XRD analyses were performed using an X’pert Pro X-ray diffractometer (PANalytical, the Netherlands) with Cu K α radiation at 40 kV and 40 mA. XRD data were collected at room temperature from 10° to 90° (2 θ ) with step increments of 0.05°. A homemade container was used to protect the powdery samples from air and moisture. The FTIR spectra were obtained with a Bruker Tensor 27 unit (Germany) in the transmission mode. A sample and potassium bromide (KBr) mixture was cold-pressed in a 1:100 weight ratio to form a pellet. The spectrum was created from 16 averaged scans with a resolution of 4 cm −1 . The Rietveld refinement was performed using RIETAN-2000 (ref. 36 ). Morphological observations The s.e.m. observations were performed with a Hitachi-S4800 microscope (Japan). The TEM observations were performed on a Hitachi-H9500 microscope (Japan) with a heating holder for the in situ Et 2 O removal and dehydrogenation processes of the [Mg(AlH 4 ) 2 (Et 2 O)] n nanorods ( Fig. 6a–h ), a FEI Tecnai G2 F20 S-TWIN electron microscope (USA) for the hydrogenated Mg(AlH 4 ) 2 nanorods ( Supplementary Fig. 8b,c ), and a JEM-2100 (JEOL, Japan) equipped with a vacuum-transfer holder (Gatan, USA) for the LiBH 4 nanobelts ( Fig. 3a,b ). Each sample was dispersed on a carbon-coated Mo grid after hand-grinding for 5 min. During the in situ TEM observations, the temperature was successively increased from room temperature to 100, 180 and 400 °C, where the sample was held for 10 min at each temperature. Here, 100 °C was used as the Et 2 O-removal temperature instead of 90 °C, as stated for the heat treatment, because the use of higher heating rates and shorter holding times during the in situ TEM increased the Et 2 O-removal temperature. EDS and SAED were employed to analyse the chemical composition and to identify the phase of the LiBH 4 nanobelts ( Fig. 3c,d ), respectively. How to cite this article: Pang, Y. et al . A mechanical-force-driven physical vapour deposition approach to fabricating complex hydride nanostructures. Nat. Commun. 5:3519 doi: 10.1038/ncomms4519 (2014).